Metal-adeninate vertices for the construction of an exceptionally porous metal-organic framework Metal-organic frameworks comprising metal-carboxylate cluster vertices and long, branched organic linkers are the most porous materials known, and therefore have attracted tremendous attention for many applications, including gas storage, separations, catalysis and drug delivery. To increase metal-organic framework porosity, the size and complexity of linkers has increased. Here we present a promising alternative strategy for constructing mesoporous metal-organic frameworks that addresses the size of the vertex rather than the length of the organic linker. This approach uses large metal-biomolecule clusters, in particular zinc-adeninate building units, as vertices to construct bio-MOF-100, an exclusively mesoporous metal-organic framework. Bio-MOF-100 exhibits a high surface area (4,300 m 2 g −1 ), one of the lowest crystal densities (0.302 g cm −3 ) and the largest metal-organic framework pore volume reported to date (4.3 cm 3 g −1 ). Periodic mesoporous materials having large pore volumes can store voluminous quantities of gas molecules (for example, CH 4 , H 2 , CO 2 and so on), accommodate large guest molecules, and they can potentially act as scaffolds for organizing nanoscale structures, including nanoparticles, polymers and proteins, into periodic assemblies [1] , [2] . The size and quantity of guest species which can diffuse into a mesoporous material depends intrinsically on the pore dimensions and pore volume. Porosity is the hallmark physical property of metal-organic frameworks (MOFs) [3] , [4] , [5] . Numerous crystalline microporous MOFs have been constructed and their porosity has been exploited for a variety of applications [6] , [7] , [8] , [9] , [10] , [11] , [12] , [13] , [14] , [15] , [16] , [17] , [18] . These materials generally consist of discrete metal cluster vertices interconnected by organic linker molecules [19] . By increasing linker length and size and targeting specific network topologies, pore metrics have been systematically increased [20] , and MOFs exhibiting some degree of mesoporosity have been reported [21] , [22] , [23] , [24] , [25] , [26] , [27] , [28] , [29] , [30] . The most common strategy employed to achieve large pore volumes involves using well-known metal-carboxylate clusters (for example, M 4 O(CO 2 ) 6 or M 2 (CO 2 ) 4 ) as building blocks and linking them together with large linkers into periodic, non-interpenetrated networks [19] . Very recently, carboxylate-linker approaches were successfully implemented to construct highly porous MOFs exhibiting both microporous and mesoporous cavities, including UMCM-1 (ref. 24 ), DUT-6 (ref. 26 ), NOTT-116 (ref. 27 ), NU-100 (ref. 29 , PCN-610 (ref. 30 ) and MOF-210 (ref. 28 ), the latter which exhibited the largest MOF pore volume ( V p =3.6 ml g −1 ) and Brunauer-Emmett-Teller (BET) surface area (6,240 m 2 g −1 ) known to date. It is expected that continued incremental increases in pore metrics will be achieved using derivations of these well-established MOF design approaches. However, using increasingly longer and complex linkers to increase pore metrics may ultimately meet limitations, because longer linkers are often more flexible, less synthetically accessible and less soluble than their commercially available counterparts. In some cases, longer linkers lead inevitably to high degrees of interpenetration and consequently low degrees of porosity [31] , [32] . An alternative and less-explored strategy to achieving high degrees of porosity in MOFs is to address the size of the metal-cluster vertex. The use of larger vertices should allow one to increase pore dimensions without using large, exotic linker molecules [33] , [34] , [35] , [36] , [37] , [38] . Here we introduce a new strategy for constructing mesoporous MOFs, which is based on constructing large metal-organic vertices, instead of metal-carboxylate cluster vertices, and periodically linking these large building units together with inexpensive, commercially available organic linkers. Using this strategy, we construct large zinc-adeninate vertices and demonstrate how these vertices can be assembled into the highly open augmented LCS net to ultimately yield an exceptionally porous material, bio-MOF-100, that exhibits exclusively mesoporous cavities and which has the largest MOF pore volume reported to date. We expect that straightforward elaboration of this strategy will lead to levels of porosity not yet achieved using the afore-described traditional MOF design strategies. Moreover, we anticipate that this and other mesoporous bio-MOFs will be potentially useful for biological applications, such as drug storage and release or for the immobilization and organization of large biomolecules [12] , [39] , [40] . Zinc-adeninate building units In recent work, we described a new class of metal-adeninate MOFs containing adenine biomolecular linkers and we showed that controlling the coordination mode of adenine can impact the structure and function of these materials [40] , [41] , [42] , [43] , [44] . Bio-MOF-1 (ref. 40 ), a representative of this class of MOFs, consists of infinite 1-D zinc-adeninate columns comprising corner-fused zinc-adeninate octahedral building units (ZABUs). These columns are interconnected by linear biphenyldicarboxylate (BPDC) linkers. Close examination of this structure reveals that the ZABUs could potentially serve as discrete metal-organic vertices for the construction of new bio-MOFs, if proper reaction conditions were identified that yielded discrete ZABUs rather than columns of fused ZABUs. Each octahedral ZABU ( Fig. 1a ) consists of eight Zn 2+ cations interconnected by four adeninates and two μ-oxo groups; monodentate BPDCs occupy the remaining coordination sites on each tetrahedral Zn 2+ (only the coordinated oxygen atoms from the BPDC linkers are shown in Fig. 1 ). The size of the ZABU necessitates that three carboxylates coordinate to each open face, resulting in a total of 12 BPDCs per unit. It is instructive to compare the size of this ZABU ( Fig. 1a ) with the size of the basic zinc-carboxylate cluster, a metal-carboxylate cluster used commonly for the construction of some of the most porous MOFs [24] , [26] , [28] . The ZABU measures 14.2 Å from top to bottom and 14.3 Å across its diameter. In comparison, the basic zinc-carboxylate cluster ( Fig. 1b ) measures ~10.5 Å in diameter. The ZABU is significantly larger than the basic zinc-carboxylate cluster: to compare, a sphere with a diameter of 14.2 Å would displace ~2.5 times more volume than a sphere with a diameter of 10.5 Å. The large size difference between the two different vertices enables one to realize the potential advantage of using metal-organic building units as vertices for constructing highly porous MOFs. Moreover, we emphasize that each ZABU connects to each neighbouring unit with three linkers instead of one, an aspect that may significantly increase the structural robustness of a framework [34] . As a MOF building block, the ZABU can be considered an intermediate between the metal-carboxylate cluster and the discrete microporous metal-organic polyhedra, which have also been linked together to form MOFs [25] , [27] , [29] , [30] , [45] . 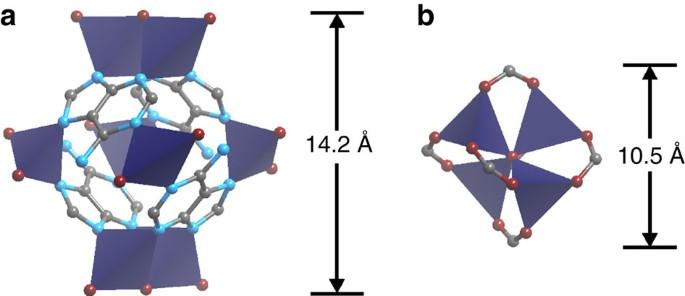Figure 1: Comparison of MOF building units. Structure and size of the zinc-adeninate building unit (ZABU) (a) compared with the structure and size of the basic zinc-carboxylate building unit (b) (Zn2+, dark blue tetrahedra; C, grey spheres; O, red spheres; N, blue spheres; H, omitted for clarity). Figure 1: Comparison of MOF building units. Structure and size of the zinc-adeninate building unit (ZABU) ( a ) compared with the structure and size of the basic zinc-carboxylate building unit ( b ) (Zn 2+ , dark blue tetrahedra; C, grey spheres; O, red spheres; N, blue spheres; H, omitted for clarity). Full size image Synthesis and single crystal X-ray analysis We expected that the discrete ZABU could serve as a vertex in an extended framework. To synthesize structures containing this discrete building unit, we heated a solution of adenine, biphenyldicarboxylic acid and zinc acetate dihydrate in N,N′ -dimethylformamide (DMF) and methanol in a capped glass vial for 24 h. This solvothermal reaction yielded colourless polyhedral block-like crystals of anionic bio-MOF-100, formulated as Zn 8 (ad) 4 (BPDC) 6 O 2 • 4Me 2 NH 2 , 49DMF, 31H 2 O. A single crystal was selected for single crystal X-ray diffraction, and it was mounted in a quartz capillary for data collection at room temperature. All attempts to find a suitable cryoprotectant to cryocool the crystals to 100 K (to reduce radiation damage to the crystal during data collection) were unsuccessful, an initial indication of the crystals' high porosity. The material crystallized in a cubic space group with cell parameters of a = b = c =69.12 Å and a cell volume of 330,230 Å 3 . The large unit cell was indicative of low crystalline density, which resulted in weak diffraction characteristics. X-ray diffraction data to 1.26 Å resolution were therefore collected on a Bruker MicroStar Cu rotating anode equipped with a charge-coupled device detector. The structure was solved by ab-initio methods using SHELXD [46] and refined by iterative cycles of restrained full-matrix least-squares techniques with Shelxl (ref. 47 ) and interactive model-building using Olex2 (ref. 48 ). The crystal structure consists of discrete ZABUs interconnected with BPDC linkers. Each ZABU ( Fig. 1a ; Supplementary Fig. S1 ) consists of eight zinc cations, four adeninate ligands and two apical oxo groups, which bridge two zinc cations together. The oxo groups were assigned based on comparing the Zn-O-Zn bond angles and Zn-O distances to similar existing structures in the Cambridge Crystallographic Database. Twelve BPDC linkers connect each cage to four neighbouring cages ( Fig. 2b ), and this connectivity is repeated periodically throughout the extended three-dimension framework, generating large cavities ( Fig. 2c ) within the structure and solvent channels measuring ~28 Å in diameter that run along [110], [101] and [011] ( Fig. 2d ; Supplementary Fig. S2 ). To our knowledge, this is the first MOF material that exclusively exhibits mesopores, an aspect that should allow for facile diffusion of large guest molecules; other reported mesoporous MOFs exhibit a combination of both micro- and mesopores [21] , [22] , [23] , [24] , [25] , [26] , [27] , [28] , [29] . The framework has a net 4-charge per formula unit. Elemental analysis was used to determine that four dimethylammonium cations, products of DMF decomposition, per formula unit reside in the pores to balance the charge. 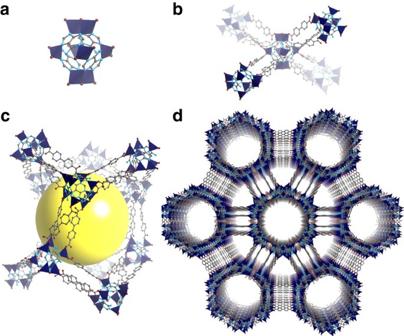Figure 2: Crystal structure of bio-MOF-100. The ZABU (a) is connected to four neighbouring ZABUs via 12 BPDC linkers (b) to generate a three-dimensional structure with large cavities (yellow sphere;c) and large channels which run along [110], [101] and [011] (note: only one channel direction shown;d) (Zn2+, dark blue tetrahedra; C, grey spheres; O, red spheres; N, blue spheres; H, omitted for clarity). Figure 2: Crystal structure of bio-MOF-100. The ZABU ( a ) is connected to four neighbouring ZABUs via 12 BPDC linkers ( b ) to generate a three-dimensional structure with large cavities (yellow sphere; c ) and large channels which run along [110], [101] and [011] (note: only one channel direction shown; d ) (Zn 2+ , dark blue tetrahedra; C, grey spheres; O, red spheres; N, blue spheres; H, omitted for clarity). Full size image It is helpful to determine the underlying network topology of bio-MOF-100 to more completely understand the structural features that lead to its highly open structure. Each ZABU adopts a distorted truncated tetrahedron topology ( Fig. 3a,b ), visualized by connecting the coordinated carboxylate oxygen atoms, which extend apically from the structural framework. Each tetrahedron unit has two angles of 100.01° and two angles of 130.73°, which are significantly distorted from those of a perfect tetrahedron (all angles 109.5°). Therefore, these building blocks do not pack into an ideal diamond lattice as one might anticipate; rather, the framework adopts an augmented LCS topology ( Fig. 3c ) [49] . As the LCS net is not a self-dual, bio-MOF-100 does not interpenetrate, a structural attribute that can naturally result in high degrees of porosity [50] , [51] . 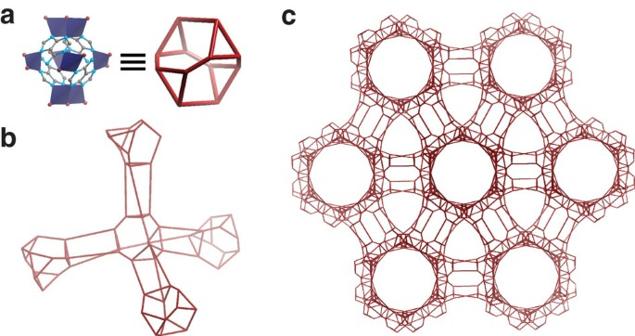Figure 3: Underlying network topology of bio-MOF-100. Each ZABU can be treated as a distorted truncated tetrahedran (a). Each truncated tetrahedran connects to four neighbouring tetrahedra (b) to generate an augmented LCS net (a-LCS;c). Figure 3: Underlying network topology of bio-MOF-100. Each ZABU can be treated as a distorted truncated tetrahedran ( a ). Each truncated tetrahedran connects to four neighbouring tetrahedra ( b ) to generate an augmented LCS net ( a -LCS; c ). Full size image The large zinc-adeninate building units and the inherent absence of interpenetration lead to a remarkably open structure with a calculated free volume of approximately 85% and one of the lowest densities reported for a crystalline material, 0.302 g cm −3 . Elemental analysis of the solvated crystals ( Fig. 4a ) reveals that the pores accommodate a total of 49 DMF and 31 water molecules per formula unit, values that were corroborated by thermogravimetric analysis (TGA) data ( Fig. 4b ). Indeed, upon heating to ~200 °C, as-synthesized bio-MOF-100 loses over 60% of its mass, which corresponds to the guest molecules. No further weight loss was observed until the material decomposes at ~350 °C. Given the rigidity of the zinc-adeninate building units and the fact that they are connected to each neighbouring unit by a total of three rigid BPDC struts, we assumed that the framework would be structurally robust and able to withstand loss of solvent guest molecules. 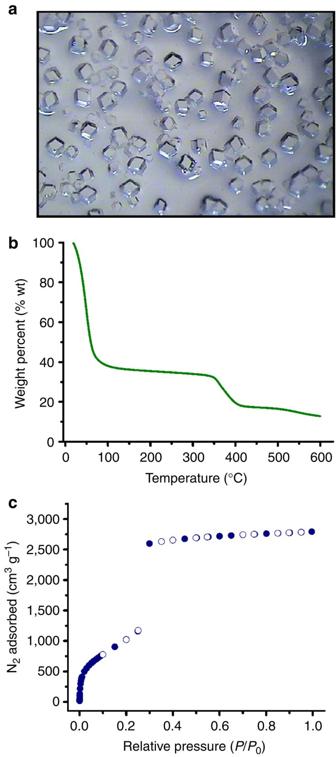Figure 4: Physical characterization of bio-MOF-100. Light microscope image of solvated bio-MOF-100 crystals (a). Thermogravimetric analysis plot of the solvated bio-MOF-100 crystals (b). N2(g) adsorption isotherm (77 K) for bio-MOF-100 (c). Figure 4: Physical characterization of bio-MOF-100. Light microscope image of solvated bio-MOF-100 crystals ( a ). Thermogravimetric analysis plot of the solvated bio-MOF-100 crystals ( b ). N 2 (g) adsorption isotherm (77 K) for bio-MOF-100 ( c ). Full size image We therefore next proceeded to measure the porosity using gas adsorption techniques. Because more traditional MOF activation methods did not yield the level of porosity that we anticipated ( Supplementary Fig. S3 ), we elected to activate the material using supercritical CO 2 exchange and subsequent evacuation, a method that has proven fruitful for activating some of the most porous MOF structures [28] , [29] , [52] , [53] . A nitrogen adsorption experiment was performed on an optimally activated sample of bio-MOF-100, and it confirmed that the structure is indeed highly porous and exhibits an isotherm consistent with mesoporosity ( Fig. 4c ). From the first plateau (~1,160 cm 3 g −1 ), we calculated a BET surface area of 4,300 m 2 g −1 (ref. 54 ). The second steep rise in the isotherm ( P / P 0 ~0.3) indicates filling of the mesopores; upon saturation (~2,800 cm 3 g −1 ), we calculated a maximum pore volume of 4.3 cm 3 g −1 . To our knowledge, this pore volume is the largest reported to date for any MOF material (~20% larger than that of MOF-210) [28] . The material remains crystalline after the gas adsorption studies, as determined by powder X-ray diffraction studies ( Supplementary Fig. S4 ). We report here our findings that large discrete metal-organic building units, in this case zinc-adeninate clusters, can be used as vertices in MOFs. When these vertices are connected using simple (and relatively short) dicarboxylate linker molecules, a new mesoporous MOF, bio-MOF-100, results, and it exhibits the largest pore volume of any known MOF material. This result points towards the utility of using metal-organic building blocks as vertices for constructing highly porous MOFs. We expect that we will be able to isolate MOFs with still larger pore volumes via straightforward elaboration of this strategy, including using longer linkers and more highly branched linkers and by constructing other large metal-biomolecule or metal-organic building units. General procedures and protocols Unless otherwise mentioned, all chemicals were purchased from Aldrich Chemical. DMF was purchased from Fisher Scientific. All purchased starting materials were used without further purification. The elemental microanalyses were performed by the University of Illinois Department of Chemistry Microanalytical Laboratory using an Exeter Analytical CE440. TGA was performed using a TGA Q500 thermal analysis system. All TGA experiments were performed under a N 2 atmosphere from 25 to 600 °C at a rate of 1 °C min −1 . Data were analysed using the TA Universal Analysis software package. Fourier transform infrared spectra were measured using a Nicolet Avatar 360 FTIR E.S.D. and KBr pellet samples. Absorptions are described as follows: very strong (vs), strong (s), medium (m), weak (w), shoulder (sh) and broad (br). Data were analysed using the Omnic Software package. X-ray powder diffraction patterns were collected using a Bruker AXS D 8 Discover powder diffractometer at 40 kV, 40 mA for Cu Kα ( λ =1.5406 Å), with a scan speed of 0.20 s per step and a step size of 0.02018°. The data were analysed for d -spacing measurements using the EVA program from the Bruker Powder Analysis Software package. The simulated powder patterns were calculated using Mercury 2.0. The purity and homogeneity of the bulk products were determined by comparison of the simulated and experimental X-ray powder diffraction patterns. Nanopure water (18 MΩ) was produced using a water purification system from Barnstead Nanopure. Synthesis and characterization of Bio-MOF-100 A stock solution of adenine (0.05 M) in DMF was prepared. Ultrasonication and heating was employed to completely dissolve adenine in DMF. A stock solution of zinc acetate dihydrate (0.05 M) and 4,4′-biphenyldicarboxylic acid (0.1 M) in DMF was prepared. Adenine stock solution (2.5 ml, 0.125 mmol), zinc acetate dihydrate stock solution (5 ml, 0.25 mmol) and 4,4′-biphenyldicarboxylic acid stock solution (2.5 ml, 0.25 mmol) were added to a 20-ml vial, then 2.5 ml of DMF, 1 ml of methanol and 0.25 ml of nanopure water were subsequently added. The vial was capped and heated at 85 °C for 24 h and then cooled to room temperature. The colourless cubic crystal products were washed with DMF (3 ml, 3×) and dried under Ar gas (30 min; yield: 0.218 g, 25.4% based on adenine). Fourier transform infrared : (KBr 4,000–400 cm −1 ): 3,341.18(br), 3,185.33(br), 2,929.70(w), 1,669.40(s), 1,607.51(s), 1,547.96(w), 1,467.74(w) 1,386.25(s), 1,255.31(w), 1,212.29(m), 1,176.27(w), 1,152.77(m), 1,097.54(m), 855.89(m) 843.48(m), 773.25(s). Elemental analysis C 259 H 501 N 73 O 106 Zn 8 =Zn 8 (ad) 4 (BPDC) 6 ,O 2 • 4Me 2 NH 2 , 49DMF, 31H 2 O. Calcd. C , 45.37; H , 7.36; N , 14.91. Found C , 45.43; H , 7.51; N , 14.84. Gas adsorption experiments by conventional activation protocol Sorption isotherm studies of Zn 8 (ad) 4 (BPDC) 6 ,O 2 • 4Me 2 NH 2 , 49DMF, 31H 2 O (bio-MOF-100) were performed volumetrically as a function of relative pressure by using the Autosorb 1 by Quantachrome. Samples of either DMF washed materials or CHCl 3 -exchanged materials were weighed using an AB54-S/FACT (Mettler Toledo) electrogravimetric balance (sensitivity 0.1 mg). Nine-mm large bulb cells (from Quantachrome) of a known weight were loaded with ~100 mg of sample for gas sorption experiments. The samples were degassed at room temperature or 100 °C for 22–24 h on degassing station until the outgas rate was no more than 3.5 mTorr min −1 . The degassed sample and sample cell were weighed precisely and then transferred back to the analyzer. The temperature of each sample for N 2 adsorption experiments was controlled by a refrigerated bath of liquid nitrogen (77 K). The N 2 adsorbates were of ultrahigh purity (UHP) grade. Gas adsorption experiments with activation via supercritical drying The general supercritical drying method is performed according to the published procedures [52] . The samples were activated with supercritical CO 2 in a Tousimis Samdri PVT-30 critical point dryer. Before drying, the DMF solvated samples were soaked in absolute ethanol (EtOH), replacing the soaking solution for 48 h, to exchange the occluded solvent for EtOH. After the EtOH exchange process was complete, the samples were placed inside the dryer and the EtOH was exchanged with CO 2(L) over a period of 8 h. During this time, the liquid CO 2 was vented under positive pressure for 5 min each hour. The rate of venting of CO 2(L) was always kept below the rate of filling so as to maintain a full drying chamber. After 8 h of venting and soaking with CO 2(L) , the chamber was sealed and the temperature was raised to 40 °C. This brought the chamber pressure to around 90 bar, that is, above the critical point of CO 2 . The chamber was vented over the course of 12–18 h. The dried samples were placed in sealed containers and stored in a desiccator. Samples of the supercritical CO 2 dried materials were weighed using an AB54-S/FACT (Mettler Toledo) electrogravimetric balance (sensitivity 0.1 mg). Nine-mm large bulb cells (from Quantachrome) of a known weight were loaded with ~50 mg of sample for gas sorption experiments. The samples were degassed at room tempertaure for 24 h on degassing station until the outgas rate was no more than 3.5 mTorr min −1 . The degassed sample and sample cell were weighed precisely and then transferred back to the analyzer. The temperature of each sample for N 2 adsorption experiments was controlled by a refrigerated bath of liquid nitrogen (77 K). The N 2 adsorbate was of ultrahigh purity (UHP) grade. Crystallographic data and structure refinement Cubic colourless crystals of approximate dimensions of 0.15×0.15×0.15 mm were mounted in a quartz capillary with some mother liquid to prevent drying out on a Bruker MicroStar Cu rotating anode equipped with Helios mirrors and a Platinum135 CCD Detector. Complete diffraction data were collected using two φ-scans of 180° with an oscillation range of 0.25° per frame at two different 2θ setting. Diffraction data to a maximum resolution of 1.26 were integrated and scaled with the Bruker Proteum software. The structure was solved by dual-space ab-inito method, as implemented in SHELXD [46] , and completed by iterative cycles of restrained full-matrix least-squares methods [55] and model analysis using Olex2 (ref. 48 ). Owing to the size and flexibility of the structure, distance restraints were applied with standard values for the adenine taken from the Nucleic Acid Database [56] . Similar distance restraints without specific target values were used for the chemically equivalent 1,2- and 1,3-distances in the 4,4-biphenyl dicarboxylic acid. All aromatic ring systems were restrained to be planar, and H-atoms were refined using a riding model. The structure was refined anisotropically with the rigid-bond restraint applied to anisotropic displacement parameters [57] , leading to chemically reasonable displacement ellipsoids as shown in Supplementary Figure S5 . The course of refinement and the weights of restraints were carefully monitored using the R free test, originally developed for protein crystallography [58] , and successfully applied to the refinement of large small-molecules [59] , [60] . The final refinement was performed against all F 2 and converged to R-factors of wR2=0.4152 and R1=0.126. A representative electron density map is shown in Supplementary Figure S6 . Further experimental and crystallographic details are summarized in Supplementary Table S1 . Accession Code: The single crystal diffraction data for bio-MOF-100 was deposited in the Cambridge Crystallographic Data Centre (CCDC) and the deposition number is CCDC 833315. How to cite this article: An, J. et al . Metal-adeninate vertices for the construction of an exceptionally porous metal-organic framework. Nat. Commun. 3:604 doi: 10.1038/ncomms1618 (2012).